Quantum coherence controls the charge separation in a prototypical artificial light-harvesting system The efficient conversion of light into electricity or chemical fuels is a fundamental challenge. In artificial photosynthetic and photovoltaic devices, this conversion is generally thought to happen on ultrafast, femto-to-picosecond timescales and to involve an incoherent electron transfer process. In some biological systems, however, there is growing evidence that the coherent motion of electronic wavepackets is an essential primary step, raising questions about the role of quantum coherence in artificial devices. Here we investigate the primary charge-transfer process in a supramolecular triad, a prototypical artificial reaction centre. Combining high time-resolution femtosecond spectroscopy and time-dependent density functional theory, we provide compelling evidence that the driving mechanism of the photoinduced current generation cycle is a correlated wavelike motion of electrons and nuclei on a timescale of few tens of femtoseconds. We highlight the fundamental role of the interface between chromophore and charge acceptor in triggering the coherent wavelike electron-hole splitting. Nature has developed sophisticated and highly efficient molecular architectures to convert sunlight into chemical energy, which is then used to nurture plants. On a microscopic level, photosynthesis consists of the following processes: light harvesting via a cascade of energy transfer steps, subsequent charge separation at the reaction centre and multi-electron catalysis. One of the key challenges for the future will be to learn how to construct artificial molecular devices enabling the harvesting of sunlight and their use either for direct electric power generation (photovoltaic approach) [1] , [2] , [3] or to drive fuel-producing photochemical reactions (photosynthetic approach) [4] , [5] . Very recently, the observation of electronic quantum coherence, that is, the wavelike motion of electrons, induced a paradigm shift [6] in describing the primary energy and charge-transfer processes both in photosynthetic bacteria [7] and in higher plants [8] , [9] , [10] . A fascinating, but so far unexplored, perspective would be to exploit such quantum coherence effects in artificial photosynthetic/photovoltaic systems to improve their performance. Here we study the dynamics of a photoexcited supramolecular carotene–porphyrin–fullerene triad [11] , [12] , which is a prototypical artificial reaction centre, by means of high time-resolution femtosecond spectroscopy and first-principles quantum-dynamical simulations. Upon photoexcitation of the porphyrin moiety, the primary event is the electron transfer to the fullerene [13] . We provide compelling evidence that the driving mechanism of this process is a correlated wavelike motion of electrons and nuclei on a timescale of few tens of femtoseconds, thus establishing the role of vibronic coherence in artificial light harvesting. Steady-state optical spectroscopy We chose a supramolecular carotene–porphyrin–fullerene triad, rather than the conceptually simpler porphyrin/fullerene dyad, as a model for exploring charge-transfer dynamics [14] , [15] because of the protective role of the carotene, suppressing photobleaching. The compound consists of a porphyrin ring acting as the primary light absorber, a fullerene electron acceptor and a carotene group serving as a hole stabilizer ( Fig. 1a ). It is known that photoexcitation of the porphyrin triggers an ultrafast electron transfer to the fullerene [13] with a charge-separation yield of up to 95% [11] . Subsequent electron transfer from the carotene to the porphyrin cation on a 100-ps timescale forms a long-lived charge-separated state, which decays back to the ground state via the radical-pair mechanism on a microsecond timescale. The optical properties of this and similar triads were carefully investigated experimentally [12] , but the microscopic mechanisms underlying the primary charge-transfer dynamics on a femtosecond timescale could not be unveiled due to insufficient time resolution. 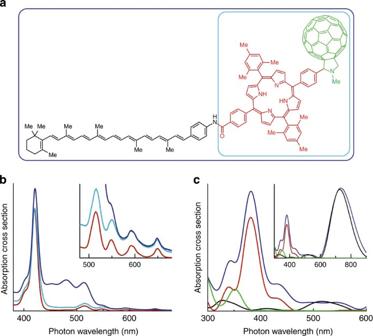Figure 1: Experimental and theoretical absorption spectroscopy. (a) Chemical structure of the carotene–porphyrin–fullerene light-harvesting triad. (b) Measured normalized absorption spectra of the triad (dark blue), a porphyrin–fullerene dyad (light blue) and an individual porphyrin unit (red) in toluene solution. The spectra have been normalized to the height of the low-energy porphyrin peaks, which are depicted magnified in the inset. (c) Absorption spectra of the triad and their individual subunits simulated by TDDFT. The triad absorption is well represented by a sum of the different subunit spectra, in accord with experiment. The porphyrin bands match reasonably well with the observed ones, once a rigid red shift of 180 meV is applied to the computed spectrum. The red shift of the main carotene peak to 730 nm reflects the excitonic quantum confinement in the quasi-one-dimensional carotene chain21. Figure 1: Experimental and theoretical absorption spectroscopy. ( a ) Chemical structure of the carotene–porphyrin–fullerene light-harvesting triad. ( b ) Measured normalized absorption spectra of the triad (dark blue), a porphyrin–fullerene dyad (light blue) and an individual porphyrin unit (red) in toluene solution. The spectra have been normalized to the height of the low-energy porphyrin peaks, which are depicted magnified in the inset. ( c ) Absorption spectra of the triad and their individual subunits simulated by TDDFT. The triad absorption is well represented by a sum of the different subunit spectra, in accord with experiment. The porphyrin bands match reasonably well with the observed ones, once a rigid red shift of 180 meV is applied to the computed spectrum. The red shift of the main carotene peak to 730 nm reflects the excitonic quantum confinement in the quasi-one-dimensional carotene chain [21] . Full size image Steady-state optical absorption spectra of the triad in toluene solution ( Fig. 1b ) show the characteristic peaks of the Soret- and the Q-band of the porphyrin moiety [16] . The broad absorption of the carotene group sets in at around 550 nm and peaks at ~510 nm. The fullerene unit induces a continuous weak absorption background throughout the visible. The assignment of these spectra is facilitated by comparison with subunit spectra of a porphyrin–fullerene dyad and of the porphyrin unit ( Fig. 1b ), and provides no evidence of charge-transfer excitations. We have calculated the absorption spectra of the triad and its subunits ( Fig. 1c ) using first-principles simulations within time-dependent density functional theory (TDDFT) [17] , [18] , [19] in Local Density Approximation. The strong Soret band and some features of the weaker Q-band of the porphyrin are well reproduced when red shifting the theoretical wavelength axis by 180 meV. The dominant carotene absorption band appears red shifted to 730 nm and is better attributed to the carotene radical cation, due to the neglect of double excitations and strong excitonic correlations [20] , [21] at this level of TDDFT. Ultrafast optical spectroscopy To probe the electron-hole splitting dynamics, we used 10-fs pulses centred around 550 nm to impulsively excite the Q-band of the porphyrin group in the triad in toluene solution. Differential transmission spectra Δ T / T ( λ , τ ) were monitored using broadband optical pulses of 7-fs duration with a spectrum depicted in Supplementary Fig. S1 . The overall time resolution of this experiment was better than 15 fs, allowing us to time-resolve the dynamics of impulsively excited vibrational modes of the triad molecule with frequencies of up to 2,000 cm −1 . Representative differential transmission spectra are shown in Supplementary Fig. S2 . These data display very rich temporal and spectral dynamics. Among the most prominent features are: (i) a slowly rising and long-lived photoinduced absorption peaking at around 575 nm, (ii) a long-lived photobleaching band centred around 523 nm and (iii) a short-lived increased transmission band extending from 540 to 580 nm. Pronounced oscillatory features are superimposed on all of these resonances, reflecting impulsively excited wavepacket dynamics of the triad supramolecule. Some of these signatures have been observed and analysed before in recent studies of photophysical properties of the individual components of the triad. The 523-nm band is understood as mainly arising from a pump-induced transient photobleaching of the absorption of the porphyrin Q-band with possible contributions from transient changes of the β-carotene S 0 ground state absorption. The photoinduced absorption band at 575 nm is well known from studies of carotenoids in solution [22] , [23] , [24] . It is assigned to excited-state absorption from the S 1 (2A g − ) carotene-state surface. Because of its broad bandwidth, the excitation pulse also couples to the S 2 state of the carotene moiety. Following a 200-fs internal conversion process, this leads to an excited-state absorption from the optically dark S 1 state of carotene. The impulsive excitation induces a large amplitude vibrational motion in the ground electronic state of the carotene moiety leading to pronounced oscillatory modulation of the Δ T / T spectra in the wavelength range between 510 and 580 nm. The impulsively excited vibrational wavepacket dynamics in β-carotene molecules are well understood and have been analysed in detail before [24] . We have analysed our data following the approach outlined in [24] and [25] , and found that primarily three ground state modes of β-carotene, with vibrational frequencies of 1003, 1155 and 1523, cm −1 , contribute to the oscillatory pattern seen in the differential transmission. These modes correspond to the methyl-rocking mode, the symmetric C-C stretch mode and the symmetric C=C stretch mode, respectively [26] . The spectral dependence of the amplitudes and phases of these vibrational modes deduced from this analysis is shown in Supplementary Fig. S3 . These parameters agree well with those deduced from the analysis of the bare carotene data, supporting the validity of this approach. To gain insight into the charge-transfer dynamics in the triad, we have subtracted these oscillations from the original data to obtain the Δ T / T spectra shown in Fig. 2a . These time-dependent spectra show two prominent features, a long-lived photobleaching of the porphyrin Q-band absorption resonance around 523 nm and a short-lived and spectrally red-shifting transient emission band in the region between 540 nm and 580 nm. The long-lived oscillatory modulation on the Q-band resonance at later times tracks impulsively excited vibrational motion in the ground state of the porphyrin moiety. 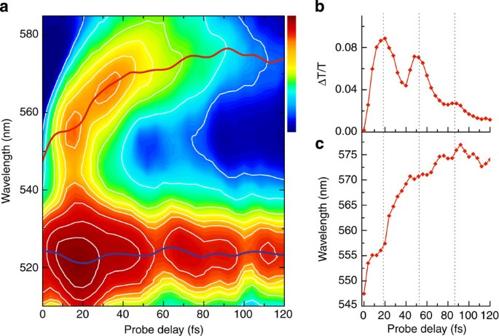Figure 2: Coherent charge-transfer dynamics in a carotene–porphyrin–fullerene triad. (a) Experimental differential transmission (ΔT/T) map as a function of time delay and probe wavelength recorded following impulsive excitation of the triad at ~550 nm. The ΔT/Tvalues are plotted on a linear colour scale extending from −0.05 to 0.12.The blue and red lines highlight the time evolution of the centre wavelengths of the porphyrin and charge-transfer bands, respectively. These centre wavelengths have been extracted from the experimental data by fitting the ΔT/Tspectra of both bands to Gaussian lineshape functions. (b,c) Temporal evolution of the ΔT/Tamplitude (b) and spectral position (c) of the charge-transfer band. The dashed lines are guides to the eye, emphasizing coherent oscillations of both amplitude and center wavelength of the charge-transfer resonance. Figure 2: Coherent charge-transfer dynamics in a carotene–porphyrin–fullerene triad. ( a ) Experimental differential transmission (Δ T / T ) map as a function of time delay and probe wavelength recorded following impulsive excitation of the triad at ~550 nm. The Δ T / T values are plotted on a linear colour scale extending from −0.05 to 0.12.The blue and red lines highlight the time evolution of the centre wavelengths of the porphyrin and charge-transfer bands, respectively. These centre wavelengths have been extracted from the experimental data by fitting the Δ T / T spectra of both bands to Gaussian lineshape functions. ( b , c ) Temporal evolution of the Δ T / T amplitude ( b ) and spectral position ( c ) of the charge-transfer band. The dashed lines are guides to the eye, emphasizing coherent oscillations of both amplitude and center wavelength of the charge-transfer resonance. Full size image A striking and novel signature of these measurements is the transient increase in transmission in the 540–580 nm region. Because of its pronounced spectral shift with time, we cannot assign it to one of the known ground state optical transitions of the individual subunits of the triad and hence we attribute it to a stimulated emission (SE) from the photoexcited electronic state. We can only track this SE for a time period of ~100 fs, which means that this emission is not coming from the final charge-separated state but rather from a transient intermediate. The data in Fig. 2 suggest temporal oscillations of not only the amplitude ( Fig. 2b ) but also the resonance wavelength ( Fig. 2c ) of this band with a period of ~30 fs. The oscillations in the resonance wavelength are not compatible with a simplified picture in which the excited electronic wavepacket moves ballistically from the donor to the acceptor state [27] . We interpret them as signature of coherent charge oscillations between donor and acceptor state. Triad dynamics on longer timescale In earlier work, evidence for the formation of a charge-separated state in porphyrin and fullerene-containing dyads and triads has been given by probing transient absorption spectra in the near-infrared region [11] , [28] . To obtain independent evidence for a photoinduced electron transfer process in the investigated CPF triad and to connect our results to earlier work, we excited a triad solution in toluene with pump pulses centred at 550 nm and with a duration of ~70 fs. The resulting changes in transmission were monitored in the near-infrared spectral range between 800 and 1,000 nm. Representative differential transmission spectra are displayed in Supplementary Fig. S4 . At all probe wavelengths, these traces display a pronounced and long-lived transient absorption signal, remaining almost constant in intensity for up to 150 ps ( Supplementary Fig. S5 ). Transient photoinduced absorption bands in the near-infrared region have also been observed in earlier studies of carotene–porphyrin–fullerene triads [11] , [28] and have been assigned to transient absorption from either the C-P + -C 60 − or the C + -P-C 60 − charge-separated state. The lifetime of the biradical C + -P-C 60 − is typically on the order of tens of nanoseconds, whereas C-P + -C 60 − decays on a nanosecond scale. To facilitate an assignment of the long-lived transient absorption in Supplementary Fig. S4 , we have performed additional transient absorption measurements, extending the probe wavelength range to beyond 1020, nm. A representative pump-probe spectrum at a delay of 30 ps is shown in Supplementary Fig. S6 . It shows a broad absorption peak at ~950 nm. Based on previous reports [28] , this peak is mostly likely dominated by the carotenoid radical anion of the C + -P-C 60 − biradical, as the extinction coefficient of the carotenoid radical exceeds that of the fullerene anion by about one order of magnitude. Irrespective of the relative contribution of the C-P + -C 60 − and the C + -P-C 60 − transient absorption to this peak, its observation is taken as a clear signature for an ultrafast electron transfer process in the investigated triad in toluene solution upon pulsed excitation at 550 nm. We find that this transient absorption is present after less than 1 ps and we take this as additional evidence that this charge transfers occurs on an ultrafast timescale. Time-dependent density functional theory We performed a detailed TDDFT quantum-dynamical description of the system to clarify the influence of coherent charge motion on the electron transfer dynamics. As no direct charge-transfer excitations are involved in the photoexcitation, the simple local approximation is expected to well describe the electron-ion dynamics during the initial charge separation. Even though the energy of the final state is likely underestimated by the approximations of the model, other important features such as the low-frequency response of the charge density were shown to be robust against the final state [29] . We have modelled the initial photoexcitation of the molecule as a sudden change in the charge density localized on the porphyrin moiety, and the resulting motion of charges and ions was tracked in space and time. In this way, we ensure that no charge is displaced to the fullerene at time zero and that we realistically mimic the Franck–Condon excitation of the porphyrin moiety occurring in the experiment. Several movies in the Supplementary Information summarize the results of the simulations ( Supplementary Movies 1–3 ). From these movies, we have deduced the time evolution of the fractional charge on the pyrrole–fullerene part of the triad by spatially integrating over the respective region of the molecule. This time evolution is presented in Fig. 3a for different simulation scenarios, by either allowing all nuclei to move freely or by locking the ionic positions in specific regions of the molecule. 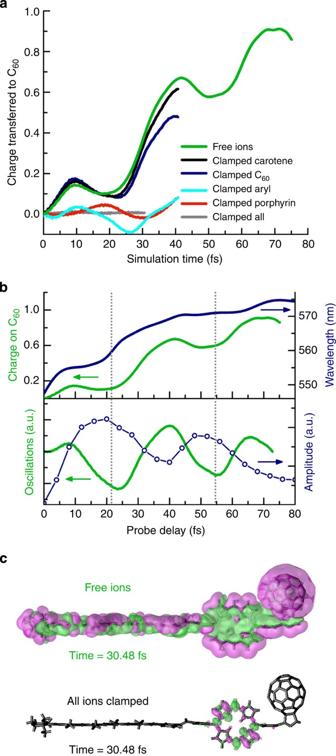Figure 3: Quantum dynamics simulations of the charge-transfer process. (a) Simulated charge transfer in the triad occurs in ~70 fs (green line). Temporal oscillations with a period of ~30 fs suggest that coherent nuclear motion drives this charge transfer. The dynamics remain unaltered when locking the positions of either the carotene (black line) or the fullerene (blue). Clamping the porphyrin (red), or only four atoms (cyan) on the connector between porphyrin and fullerene fully suppresses the charge accumulation. (b) Correlation between temporal oscillations in the simulated transferred charge (green lines, in lower panel the slow exponential rise was subtracted) and in the resonance wavelength (blue, upper panel) and the amplitude (blue, lower panel) of the differential transmission spectrum of the charge-transfer band. This correlation is evidence for the coherent motion of electrons and nuclei during the charge transfer. (c) Snapshots of the photoinduced change in charge density at a time delay of 30.48 fs for the free triad (upper panel) and with all atoms clamped. Magenta indicates an increase in electronic charge density, whereas a decrease is shown in green. a.u., arbitrary units. Figure 3: Quantum dynamics simulations of the charge-transfer process. ( a ) Simulated charge transfer in the triad occurs in ~70 fs (green line). Temporal oscillations with a period of ~30 fs suggest that coherent nuclear motion drives this charge transfer. The dynamics remain unaltered when locking the positions of either the carotene (black line) or the fullerene (blue). Clamping the porphyrin (red), or only four atoms (cyan) on the connector between porphyrin and fullerene fully suppresses the charge accumulation. ( b ) Correlation between temporal oscillations in the simulated transferred charge (green lines, in lower panel the slow exponential rise was subtracted) and in the resonance wavelength (blue, upper panel) and the amplitude (blue, lower panel) of the differential transmission spectrum of the charge-transfer band. This correlation is evidence for the coherent motion of electrons and nuclei during the charge transfer. ( c ) Snapshots of the photoinduced change in charge density at a time delay of 30.48 fs for the free triad (upper panel) and with all atoms clamped. Magenta indicates an increase in electronic charge density, whereas a decrease is shown in green. a.u., arbitrary units. Full size image The quantum dynamics simulations suggest a rapid and almost complete charge flow to the fullerene moiety within ~70 fs ( Figs 3a ) when allowing all ions to freely move during the charge-transfer process. On this timescale, the launched electronic wavepacket oscillates a few times, with a period of 30 fs, back and forth between the carotene–porphyrin group and the fullerene moiety. Both the timescale of the charge build-up and the oscillation period of the electronic wavepacket agree well with the experimentally observed values ( Fig. 3b ). The agreement becomes even more striking by comparing Fourier spectra of the simulated charge-transfer dynamics ( Fig. 4a ) to those of the experimental amplitude and resonance wavelength dynamics ( Fig. 4b ). For both the experimental amplitude data and the simulated charge dynamics, the spectra reveal a distinct peak at ~1,000 cm −1 , corresponding to an oscillation period of 33 fs. Even the Fourier transform of the strongly red-shifting resonance wavelength (inset in Fig. 4b ) reveals a dominant resonance at 930 cm −1 (36 fs), although the weak oscillatory contrast on the time-resolved data in Fig. 2 precludes a quantitative assignment of the spectrum. Within the accuracy of the presented results, the experimentally observed and simulated oscillation period of ~30 fs is reasonably close to that of the carbon backbone vibrations, with a frequency of the dominant excited-state C-C stretch motion of 1,230 cm −1 ( [30] ). This suggests that nuclear motion delocalized across the porphyrin/fullerene region drives the charge transfer. This conclusion is strongly supported by the small change in the transfer dynamics observed in the simulations when the positions of either the carotene or the fullerene ions are blocked ( Fig. 3a ). On the other hand, even minor changes of the nuclear vibrations in the porphyrin/linker/fullerene region of the molecule can greatly influence the charge flow. Upon locking the porphyrin ions or only four atoms on the aryl-ring connecting porphyrin and fullerene, charge accumulation on the fullerene is greatly suppressed ( Fig. 3a ), whereas the coherent charge oscillations at the backbone vibrational frequency still persist. Fixing the position of all ions, on the other hand, suppresses both charge oscillation and accumulation. In general, we find that the TDDFT calculations provide an estimate of the overall timescale of the charge-transfer process of ~70 fs, which is in quite good agreement with that deduced from the shift in resonance wavelength of the charge-transfer band seen in Fig. 2b . Also the period of the predicted charge oscillations of ~30 fs agrees well with our experimental measurements. Remaining differences in the phase of those oscillatory patterns ( Fig. 3b ) likely reflect the different excitation and probing conditions in experiment and theory and possible small uncertainties (a few femtoseconds) in the measurement of the experimental time zero. Both experimental and theoretical results suggest that the charge degrees of freedom in our molecule are strongly coupled to the carbon backbone vibration. A detailed understanding of this coupling mechanism requires a refined analysis of the potential energy surfaces of this large molecule, specifically of conformational changes between ground and excited electronic states. Such information is beyond the scope of the mean-field Ehrenfest approach presented here. A deeper quantum-chemical analysis of the coupling mechanism is currently underway. 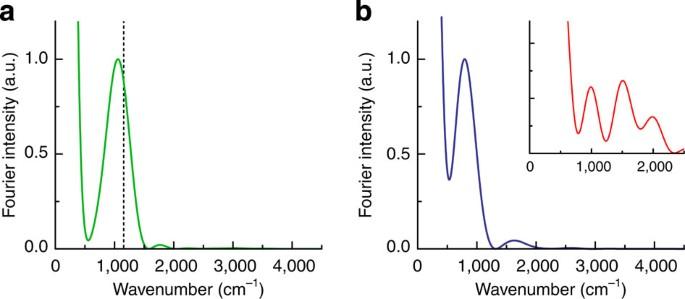Figure 4: Fourier intensity spectra of the charge-transfer dynamics in a carotene–porphyrin–fullerene triad. Fourier intensity spectrum of the simulated charge-transfer dynamics towards the fullerene (a, data taken fromFig. 3a), showing a resonance at 1060±190 cm−1, and of the temporal variation of the (ΔT/T) amplitude of the charge-transfer band (b, data taken fromFig. 2b) with a resonance at 940±100 cm−1, corresponding to an oscillation period of 35 fs. The inset in panelbdisplays the Fourier intensity spectrum of the observed temporal red shift of the charge-transfer band (data taken fromFig. 2c), revealing a dominant peak at 930±90 cm−1. The broad shoulder below 820 cm−1reflects the pronounced shift in resonance wavelength inFig. 2con a 100-fs-timescale. The black dashed line indicates the frequency of the carotene symmetric C-C stretch mode at 1155, cm−1. The data were padded to 0 with exponentially decaying tails at both sides before Fourier transformation. We take the fact that the main oscillatory resonance in the Fourier transforms of both the time-dependent amplitude and resonance wavelength peaks around 940 cm−1, as experimental signature that the differential transmission spectra of the charge-transfer band are modulated by an oscillatory wavepacket motion with a period of ~30 fs. Within our signal-to-noise ratio, this matches well with the oscillation period seen in the simulated charge-transfer dynamics, reflecting the nuclear motion of the carbon backbone. a.u., arbitrary units. Figure 4: Fourier intensity spectra of the charge-transfer dynamics in a carotene–porphyrin–fullerene triad. Fourier intensity spectrum of the simulated charge-transfer dynamics towards the fullerene ( a , data taken from Fig. 3a ), showing a resonance at 1060±190 cm −1 , and of the temporal variation of the (Δ T / T ) amplitude of the charge-transfer band ( b , data taken from Fig. 2b ) with a resonance at 940±100 cm −1 , corresponding to an oscillation period of 35 fs. The inset in panel b displays the Fourier intensity spectrum of the observed temporal red shift of the charge-transfer band (data taken from Fig. 2c ), revealing a dominant peak at 930±90 cm −1 . The broad shoulder below 820 cm −1 reflects the pronounced shift in resonance wavelength in Fig. 2c on a 100-fs-timescale. The black dashed line indicates the frequency of the carotene symmetric C-C stretch mode at 1155, cm −1 . The data were padded to 0 with exponentially decaying tails at both sides before Fourier transformation. We take the fact that the main oscillatory resonance in the Fourier transforms of both the time-dependent amplitude and resonance wavelength peaks around 940 cm −1 , as experimental signature that the differential transmission spectra of the charge-transfer band are modulated by an oscillatory wavepacket motion with a period of ~30 fs. Within our signal-to-noise ratio, this matches well with the oscillation period seen in the simulated charge-transfer dynamics, reflecting the nuclear motion of the carbon backbone. a.u., arbitrary units. Full size image Our results shed new light onto the microscopic origin of the experimentally observed charge-transfer dynamics. Clearly, a simplified, often assumed static picture of molecular level alignment [31] , [32] is not sufficient to describe the first steps of the charge-separation process [14] , [15] . Instead a coherent dynamical picture emerges as the correct physical framework for the splitting of the photogenerated electron-hole pair. Optical excitation launches an electronic wavepacket onto the excited-state surface of the absorber. This simultaneously induces coherent nuclear motion of the carbon backbone and charge oscillations between the absorber and the acceptor. The transient charge generation on the acceptor leads to a gradual rearrangement of the molecular geometry and a concomitant time-dependent change of the acceptor potential energy surface. This dynamical geometric rearrangement is necessary to stabilize the charge accumulation on the acceptor and gives rise to the experimentally observed red shift of the SE spectrum. Hence, it is the concerted coherent motion of strongly coupled electrons and ions that drives the charge separation in this triad, while the surrounding environment, specifically the polarity of the solvent, apparently has a less important role, in accordance with previous observations [11] . Taken together, our experimental and theoretical data provide compelling evidence that the correlated, quantum-coherent motion of ions and electrons not only governs the first steps of the photoinduced electron dynamics but also the yield of the charge separation in this prototypical artificial light-harvesting system, in stark contrast to prevailing statistical models for electron transfer reactions. Specifically our results suggest that the carbon backbone motion promotes coherent charge oscillations, whereas rapid geometric rearrangements of the donor–acceptor structure are crucial in stabilizing the separated charges. This implies that not only the geometric and electronic structure of a photovoltaic material but also the flexibility of its molecular structure, and in particular of the donor and donor–acceptor linking group, is an important parameter for optimizing its yield. It seems interesting to explore this new optimization parameter and to further test interface quantum coherence effects in technologically relevant devices to improve their performance. Chemical synthesis For the synthesis of the triad, the three different modules, that is, the porphyrin-, the fullerene- and the carotenoid part were prepared separately and finally linked together by a 1,3-dipolar cycloaddition and amide formation according to a literature protocol [11] . The formation of the porphyrin part started from pyrrole and mesitylaldehyde. The resulting dipyrromethane was condensed with methyl 4-formylbenzoate to form the symmetric 5,15-dimesityl-10,20-bis[4-(methoxycarbonyl)phenyl]porphyrin by a known procedure [33] , [34] , [35] . Several functional group interconversions [36] led to a porphyrin with a carboxylic acid at the western end (cf. Fig. 1a ), which is needed for the already mentioned final amidation step. A carbaldehyde group was implemented at the eastern end, which was converted with fullerene in a 1,3-dipolar cycloaddition of an azomethine ylide (prepared from N -methylglycine in situ ) to form the porphyrin–fullerene module of the triad [37] . The carotenoid part of the triad had been prepared before, but the established synthesis [38] turned out to give unsatisfactory results. Therefore, a new two-step synthesis was developed, starting from 4-nitrobenzyltriphenylphosphoniumbromide, which was reduced to the aniline in the first step with H 2 and Pd/C (ref. 39 ). The second step was a Wittig reaction with apocarotinal to form the desired carotenoid. Experimental The femtosecond transient absorption spectrometer starts with a regeneratively amplified mode-locked Ti:Sapphire laser system (Clark-MXR model CPA-1) delivering pulses with 150 fs duration, 500 μJ energy, at 1 kHz repetition rate and 780 nm central wavelength. The system drives three independent non-collinear optical parametric amplifiers (NOPAs) [40] , which generate the pump and the probe pulses for the time-resolved experiments. The first NOPA (NOPA1) generates broadband visible pump pulses at 550 nm, compressed to 10 fs duration by multiple bounces on custom-designed chirped mirrors; these pulses are used to resonantly excite the Q-band of the porphyrin. The second NOPA (NOPA2) generates broadband pulses in the near-infrared frequency range (from 820 nm to 1020, nm), which are compressed by a Brewster-cut fused-silica prism pair. The third NOPA (NOPA3) generates broadband visible pulses (500–700 nm range) compressed to 7 fs duration by a pair of chirped mirrors and used to probe the transient absorption of the triad. Supplementary Figure S1 shows typical spectra from the three NOPAs. The sample is contained in a cuvette with 250-μm-thick fused-silica windows and ~300-μm optical path. After the sample, the probe beam is selected by an iris and focused onto the entrance slit of a spectrometer equipped with a 1024-pixel linear photodiode array and electronics specially designed for fast read-out times and low noise [41] . The spectral resolution of the spectrograph (~2 nm) is largely sufficient for our experiments. A fast analog-to-digital conversion card with a 16-bit resolution enables single-shot recording of the probe spectrum at the full 1-kHz repetition rate. By recording pump-on and pump-off probe spectra, one can calculate the differential transmission (Δ T / T ) spectrum at the specific probe delay τ as: By repeating this procedure for a few 100 ms and averaging the resulting signals, it is thus possible to achieve a high enough signal-to-noise ratio. By moving the translation stage, we record Δ T / T spectra at different probe delays, thus obtaining a complete two-dimensional (2D) map: Δ T / T =Δ T / T ( λ , τ ). Theoretical TDDFT simulations of the coupled electron and ion dynamics of the triad were carried out in gas phase on a molecule without porphyrin side groups at the Local Density Approximation level using the Perdew–Zunger correlation functional with the open-source code octopus [17] . The system was described on a real space grid with a 0.2-Å spacing and propagated in time for 72.8 fs in total, with a time step of 1.7 as. The time propagator was approximated by a fourth-order Taylor expansion [17] . The core electrons were represented via Troullier–Martins pseudopotentials (for s , p and d components, the cutoff radii of the pseudopotentials are 1.25 Bohr for hydrogen atoms, 1.47 Bohr for carbon atoms, and 1.39 Bohr for nitrogen and oxygen atoms), and the interpolating scaling functions method [42] was used to efficiently solve the Poisson equation in the calculation of the Hartree potential. Time-dependent optical spectra were calculated by propagating the state of the system for an additional 18.6 fs after the charge density underwent an impulsive perturbation at given times. The orbitals were propagated with the time-symmetry-enforced method [43] using a Lanczos algorithm to evaluate the propagation operator with a time step of 7.9 as, resulting in a spectral range window for the dynamical polarizability of at least 8 eV. In all present calculations, the nuclei are considered as classical particles, but the ion-electron dynamics is treated with an Ehrenfest scheme controlled at the electronic propagation time-step [44] , [45] . This approximation is expected to adequately describe the electron-ion dynamics during the initial charge-separation process even though the energetics of the final state are evidently affected by the approximations introduced at this level of DFT. The TDDFT calculations predict the time-dependent evolution of the changes in the local electron charge density n ( r , τ ) within the triad upon photoexcitation. In our calculations, we have modelled the system state at time τ =0 as a single-particle excitation between those triad electronic states whose charge configuration resembles most closely that of the isolated porphyrin’s HOMO and LUMO levels. It corresponds to an instantaneous change in the charge density, which is localized on the porphyrin moiety. This model reflects the fully localized nature of the optical excitation. In agreement with the experimental evidence that no charge-transfer excitations are observed in the optical spectrum of the triad, no charge separation is implied in the initial excitation, whereas it is instead observed as the result of the concerted electron and nuclear time evolution from the initial excited state. The resulting evolution in the charge density is then tracked as a function of the time delay τ after excitation. To visualize these dynamics, we have created movies of the time-dependent change in local electron charge density δ n ( r , τ )= n ( r , τ )− n ( r , 0) by computing the difference between the charge density at delay τ and that at time zero. We have also calculated time-resolved photoabsorption cross sections at certain time delays τ after excitation. The spectra are shown in Supplementary Fig. S7 . To deduce these spectra, additional TDDFT simulations are performed, impulsively re-exciting the system at the chosen delay time τ i and computing the propagation for an additional 18.6 fs at time steps of 1.7 as. These spectra are calculated by taking as an initial condition not only the nuclear geometry at time τ i but also the excited-state electronic charge density n ( r , τ i ) reached by the molecule during its initial, free time evolution. How to cite this article: Rozzi, C. A. et al. Quantum coherence controls the charge separation in a prototypical artificial light-harvesting system. Nat. Commun. 4:1602 doi: 10.1038/ncomms2603 (2013).